Ultrafast fluorescence imagingin vivowith conjugated polymer fluorophores in the second near-infrared window In vivo fluorescence imaging in the second near-infrared window (1.0–1.7 μm) can afford deep tissue penetration and high spatial resolution, owing to the reduced scattering of long-wavelength photons. Here we synthesize a series of low-bandgap donor/acceptor copolymers with tunable emission wavelengths of 1,050–1,350 nm in this window. Non-covalent functionalization with phospholipid–polyethylene glycol results in water-soluble and biocompatible polymeric nanoparticles, allowing for live cell molecular imaging at >1,000 nm with polymer fluorophores for the first time. Importantly, the high quantum yield of the polymer allows for in vivo , deep-tissue and ultrafast imaging of mouse arterial blood flow with an unprecedented frame rate of >25 frames per second. The high time-resolution results in spatially and time resolved imaging of the blood flow pattern in cardiogram waveform over a single cardiac cycle (~200 ms) of a mouse, which has not been observed with fluorescence imaging in this window before. I n vivo biological imaging in the second near-infrared window (NIR-II, 1.0–1.7 μm) has attracted much interest recently [1] , [2] , [3] , [4] , [5] , [6] , [7] , [8] owing to salient advantages over imaging in the visible (400–750 nm) and the conventional near-infrared (NIR, 750–900 nm) regions. Detecting longer-wavelength photons in the NIR-II affords reduced photon scattering in biological tissues accompanied by lower autofluorescence, leading to higher spatial resolution at deeper tissue penetration depths [9] . To date, single-walled carbon nanotubes (SWNTs) [1] , [2] , [3] , [10] , [11] , [12] , [13] , [14] , semiconducting quantum dots (QDs) [6] , [7] , [15] , [16] , [17] , rare-earth doped nanoparticles [8] and nanoparticles made of small organic molecules [18] are fluorophores used for fluorescence imaging in the NIR-II region. These NIR-II agents can be functionalized with hydrophilic molecules to afford biocompatibility for intravenous administration and can be gradually cleared out from the body without obvious acute or chronic toxicity in animal studies [16] , [19] , [20] . However, shortcomings of existing NIR-II fluorophores include relatively low fluorescence quantum yield [1] , [8] , [21] , unfavourably short emission wavelength [18] and potential toxicity due to heavy metals in QDs [6] , [7] , [15] , [16] , [17] . A much wider range of fluorophores could be developed to tackle these problems. An ideal fluorophore developed for NIR-II biological imaging should allow for tunable excitation and emission wavelengths in the >1,000-nm NIR-II region with a high fluorescence quantum yield and high biocompatibility. Here we report the synthesis of conjugated polymers with intrinsic fluorescence >1,000 nm through donor–acceptor (D–A) alternating copolymerization, an effective way of synthesizing polymers with tunable bandgap energy in the NIR and at even longer-wavelength regions [22] , [23] , [24] , [25] , [26] , [27] , [28] , [29] . By copolymerization of an electron-donating monomer benzo[1,2-b:3,4-b′]difuran and an electron-withdrawing monomer fluorothieno-[3,4-b]thiophene, we derive a brightly fluorescent copolymer, poly(benzo[1,2-b:3,4-b′]difuran- alt -fluorothieno-[3,4-b]thiophene) (named ‘pDA’) with fluorescence emission at ~1,050 nm with a large Stokes shift of~400 nm and a high fluorescence quantum yield of ~1.7%, much higher than the quantum yield of typical carbon nanotubes (~0.4%) used previously [3] . We non-covalently functionalize the polymer with a PEGylated surfactant to afford water solubility and biocompatibility. We successfully tune the emission wavelength of the conjugated polymer fluorophores from 1,050 to 1,350 nm, and demonstrate the first in vitro and in vivo biological imaging in the >1,000-nm window using conjugated polymer fluorophores. Synthesis of NIR-II fluorescent pDA-PEG nanoparticles The pDA polymer was synthesized through a copolymerization reaction of two monomers, 1-(4,6-dibromo-3-fluorothieno[3,4-b]thiophen-2-yl)nonan-1-one and 2, 6-bis(trimethyltin)-4,8-bis (2-ethylhexyloxy)benzo[1,2-b;3,4-b′]difuran [26] . Fluorine was introduced into the thienothiophene unit to tune the fluorescence to long wavelengths ( Fig. 1 ). The pDA polymer was characterized by 1 H NMR spectroscopy (see Methods and Supplementary Figs 1–4 ) and gel permeation chromatography. The average molecular weight ( M n ) of the polymer was ~16 kDa (see Methods and Supplementary Fig. 5 ). We dissolved the as-made pDA polymer in tetrahydrofuran (THF) and then mixed it with an aqueous solution of a biocompatible surfactant of PEGylated phospholipid (DSPE-mPEG (5 kDa)) [1] , [3] , [19] (see Methods). The mixture was dialysed against water to remove THF, resulting in a stable aqueous solution of supramolecular conjugate comprising the hydrophobic core of pDA and the hydrophilic shell of DSPE-mPEG coating ( Fig. 2a ; named as pDA-PEG). 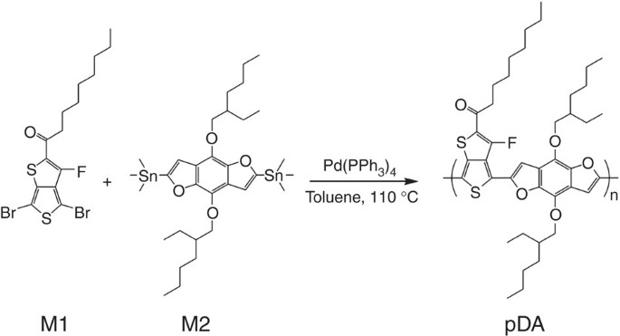Figure 1: Scheme for the Synthesis of pDA Polymer. This scheme shows the chemical structures of the two monomers M1 and M2, along with the structure of the pDA polymer, poly(benzo[1,2-b:3,4-b']difuran-alt-fluorothieno-[3,4-b]thiophene). Figure 1: Scheme for the Synthesis of pDA Polymer. This scheme shows the chemical structures of the two monomers M1 and M2, along with the structure of the pDA polymer, poly(benzo[1,2-b:3,4-b']difuran- alt -fluorothieno-[3,4-b]thiophene). 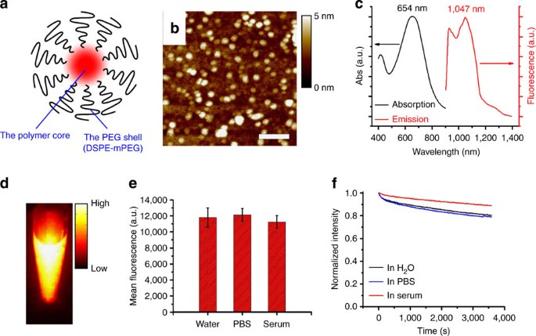Figure 2: Characterizations of pDA-PEG nanoparticle. (a) A schematic of the pDA-PEG nanoparticle showing a hydrophobic polymer core and a hydrophilic PEG shell. (b) A typical AFM image of pDA-PEG nanoparticles deposited on a silicon substrate. Owing to the effect of tip size convolution in AFM66, the height measurement from the AFM micrograph, rather than the lateral size measurement, was used to measure the size of the nanoparticles deposited on the substrate. The lateral scale bar inbindicates 100 nm. (c) Absorption and emission spectra of pDA-PEG, featuring a large Stokes shift of ~400 nm. (d) An NIR-II fluorescence image of an aqueous solution of pDA-PEG taken in the range of 1.0–1.7 μm NIR-II window under an excitation of 808 nm. (e) Fluorescence stability of pDA-PEG in different media including water, PBS and serum. The error bars were obtained by taking the s.d. of all pixel intensities within an region of interest (ROI) covering the solution in the 1-mm cuvette, as shown inSupplementary Fig. 8. (f) Photostability curves of pDA-PEG in water, PBS and serum under continuous 808-nm illumination. pDA-PEG in serum exhibits the lowest degree of photobleaching (<10%) among the three. Full size image Figure 2: Characterizations of pDA-PEG nanoparticle. ( a ) A schematic of the pDA-PEG nanoparticle showing a hydrophobic polymer core and a hydrophilic PEG shell. ( b ) A typical AFM image of pDA-PEG nanoparticles deposited on a silicon substrate. Owing to the effect of tip size convolution in AFM [66] , the height measurement from the AFM micrograph, rather than the lateral size measurement, was used to measure the size of the nanoparticles deposited on the substrate. The lateral scale bar in b indicates 100 nm. ( c ) Absorption and emission spectra of pDA-PEG, featuring a large Stokes shift of ~400 nm. ( d ) An NIR-II fluorescence image of an aqueous solution of pDA-PEG taken in the range of 1.0–1.7 μm NIR-II window under an excitation of 808 nm. ( e ) Fluorescence stability of pDA-PEG in different media including water, PBS and serum. The error bars were obtained by taking the s.d. of all pixel intensities within an region of interest (ROI) covering the solution in the 1-mm cuvette, as shown in Supplementary Fig. 8 . ( f ) Photostability curves of pDA-PEG in water, PBS and serum under continuous 808-nm illumination. pDA-PEG in serum exhibits the lowest degree of photobleaching (<10%) among the three. Full size image Atomic force microscopy (AFM) revealed the size distribution of pDA-PEG nanoparticles ( Fig. 2b ) with an average size of 2.9 nm when dried on a silicon surface ( Supplementary Fig. 6 ). The UV–vis-NIR absorption spectrum of the as-made pDA-PEG solution in water exhibited an absorption peak at 654 nm, while the fluorescence emission spectrum showed a main emission peak at 1,047 nm, suggesting a large Stokes shift of ~400 nm ( Fig. 2c ). The pDA copolymer has been reported to have red-shifted absorption and emission compared with the corresponding homopolymers because of the formation of a charge-transfer structure between the electron donor and acceptor units [26] , [27] , [30] . The fluorescence quantum yield of pDA-PEG in a solution ( Fig. 2d ) under an excitation of 808 nm was ~1.7%, measured against a standard IR-26 dye as a reference [31] , [32] ( Supplementary Fig. 7a–f , where the excitation of 808 nm was intentionally chosen to balance absorption and scattering to afford maximum penetration depth of excitation light for in vivo imaging). The quantum yield was much higher than that of typical nanotubes (~0.4%; Supplementary Fig. 7g–i ). The pDA-PEG exhibited high photostability in phosphate-buffered saline (PBS) and fetal bovine serum with negligible decay under continuous excitation for 1 h ( Fig. 2e,f and Supplementary Fig. 8 ). These results suggested pDA-PEG as an aqueous soluble, photo-stable and high brightness NIR-II fluorescent agent suited for biological imaging. Molecular imaging of cells with pDA-PEG in NIR-II We investigated pDA-PEG as a fluorescent label capable of targeting specific molecules on cell surfaces for performing molecular imaging of cancer cells through functionalization of pDA with targeting ligands. We made pDA-PEG-NH 2 using an amine-terminated phospholipid surfactant, DSPE-PEG-NH 2 (refs 33 , 34 ) Cetuximab (Erbitux) antibodies were then thiolated and conjugated to pDA-PEG-NH 2 via standard crosslinking reaction between the -NH 2 groups on the polymer and -SH groups on the thiolated antibody (see Methods). Then the pDA-PEG-Erbitux was applied to target the epidermal growth factor receptors (EGFRs) on the cell membranes of EGFR-positive breast tumour MDA-MB-468 cells, while the EGFR-negative brain tumour U87-MG cells were used as a negative control [15] . Cell imaging in NIR-II detected >1,000-nm fluorescence of pDA-PEG-Erbitux ( Fig. 3 ) selectively on the EGFR-positive MDA-MB-468 cells and not on the negative U87-MG cells, showing a positive/negative ratio of ~5.8. Thus, the pDA-PEG was made into an NIR-II fluorescent agent capable of recognizing and staining live cells with molecular specificity. This opened up the possibility of molecular imaging with conjugated copolymers in vitro and in vivo , which would not be attainable by structural imaging techniques such as ultrasound and optical coherence tomography (OCT) [35] , [36] . 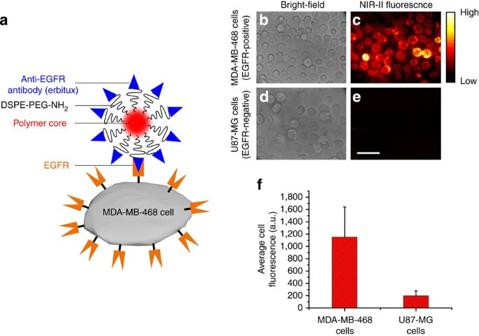Figure 3: Molecular cell imaging with pDA-PEG-Erbitux. (a) A schematic showing the structure of pDA-PEG-Erbitux bioconjugate, where the anti-EGFR antibody (Erbitux) selectively targets EGFR on the cell membrane of an MDA-MB-468 cell. (b,c) White-light (b) and NIR-II (c) fluorescence images of EGFR-positive MDA-MB-468 cells incubated with the pDA-PEG-Erbitux bioconjugate, showing positive staining of cells. (d,e) White-light (d) and NIR-II (e) fluorescence images of EGFR-negative U87-MG cells incubated with the pDA-PEG-Erbitux bioconjugate, without obvious staining of the cells. The scale bar ineindicates 40 μm, which applies to all images shown inb–e. (f) Average NIR-II fluorescence of EGFR-positive MDA-MB-468 cells and negative U87-MG cells, showing a positive/negative ratio of ~5.8. The error bars infwere obtained by taking the s.d. of average fluorescence intensity from 20 cells in each NIR-II fluorescence image. Figure 3: Molecular cell imaging with pDA-PEG-Erbitux. ( a ) A schematic showing the structure of pDA-PEG-Erbitux bioconjugate, where the anti-EGFR antibody (Erbitux) selectively targets EGFR on the cell membrane of an MDA-MB-468 cell. ( b , c ) White-light ( b ) and NIR-II ( c ) fluorescence images of EGFR-positive MDA-MB-468 cells incubated with the pDA-PEG-Erbitux bioconjugate, showing positive staining of cells. ( d , e ) White-light ( d ) and NIR-II ( e ) fluorescence images of EGFR-negative U87-MG cells incubated with the pDA-PEG-Erbitux bioconjugate, without obvious staining of the cells. The scale bar in e indicates 40 μm, which applies to all images shown in b – e . ( f ) Average NIR-II fluorescence of EGFR-positive MDA-MB-468 cells and negative U87-MG cells, showing a positive/negative ratio of ~5.8. The error bars in f were obtained by taking the s.d. of average fluorescence intensity from 20 cells in each NIR-II fluorescence image. Full size image Ultrafast blood flow tracking with pDA-PEG in NIR-II Next, we performed in vivo mouse blood vessel imaging by detecting the >1,000-nm fluorescence of intravenously injected pDA-PEG solutions. Owing to the bright fluorescence of pDA-PEG with a fourfold higher quantum yield (1.7%) than nanotube fluorophores [3] (quantum yield ~0.4%), we were able to dynamically image and track real-time arterial blood flow in the mouse hindlimb with a much shorter exposure time (~20 ms) than previously possible (~100 ms) in the NIR-II window [3] . Immediately following a tail vein injection of 200 μl solution of pDA-PEG, we performed video-rate imaging of the left hindlimb of a mouse in the supine position with an ultrafast frame rate of 25.6 frames per second (f.p.s.) compared with the previously achievable 5.3 f.p.s. (ref. 3 ). Such a high imaging speed enabled clear observation of the fast-moving flow front in the femoral artery as the NIR-II emitting pDA-PEG entered the hindlimb ( Supplementary Movie 1 and Fig. 4a ). The average femoral blood flow velocity was quantified by plotting the distance travelled by the flow front as a function of time, showing an overall linear increase with an average blood velocity of 4.36 cm s −1 ( Fig. 4b ), consistent with measurement using ultrasound (4~7 cm s −1 ) (ref. 3 ). This represented the first in vivo blood flow velocity measurement by direct tracking through real-space imaging of fast-moving flow front on the millisecond scale using NIR-II fluorescence. 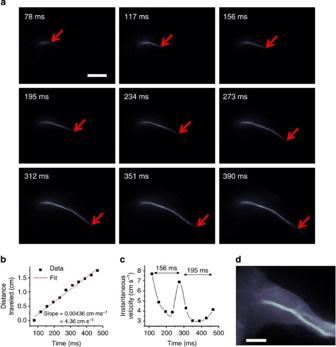Figure 4: Ultrafast NIR-II imaging of arterial blood flow. (a) A time course of NIR-II fluorescence images of a mouse hindlimb immediately following intravenous injection of pDA-PEG, showing the blood flow front moving inside the femoral artery (indicated by red arrows). The frame rate of imaging is 25.6 f.p.s. with an exposure time of 20 ms and an instrument overhead time of 19 ms. (b) A plot of the distance travelled by the blood flow front as a function of time. The linear fit reveals an average blood velocity of 4.36 cm s−1in the femoral artery. (c) A plot of instantaneous velocity (derived by dividing flow front travelled distance between two consecutive frames by the time interval of 39 ms) as a function of time, revealing periodic changes of instantaneous velocity corresponding to cardiac cycles. (d) An NIR-II fluorescence image of the same mouse hindlimb after full perfusion of pDA-PEG-containing blood into the hindlimb, upon which the fluorescence intensity in the hindlimb became unchanging. The scale bars ina,dindicate 5 mm. Figure 4: Ultrafast NIR-II imaging of arterial blood flow. ( a ) A time course of NIR-II fluorescence images of a mouse hindlimb immediately following intravenous injection of pDA-PEG, showing the blood flow front moving inside the femoral artery (indicated by red arrows). The frame rate of imaging is 25.6 f.p.s. with an exposure time of 20 ms and an instrument overhead time of 19 ms. ( b ) A plot of the distance travelled by the blood flow front as a function of time. The linear fit reveals an average blood velocity of 4.36 cm s −1 in the femoral artery. ( c ) A plot of instantaneous velocity (derived by dividing flow front travelled distance between two consecutive frames by the time interval of 39 ms) as a function of time, revealing periodic changes of instantaneous velocity corresponding to cardiac cycles. ( d ) An NIR-II fluorescence image of the same mouse hindlimb after full perfusion of pDA-PEG-containing blood into the hindlimb, upon which the fluorescence intensity in the hindlimb became unchanging. The scale bars in a , d indicate 5 mm. Full size image Interestingly, high time-resolution analysis of blood flow front position versus time revealed periodic variations in instantaneous velocity over time with a period of 150–200 ms, showing oscillations between the highest instantaneous blood velocity of ~8 cm s −1 and the lowest blood velocity of ~2 cm s −1 , corresponding to the ventricular ejection (systolic) and ventricular relaxation (diastolic) phases, respectively, of a single cardiac cycle ( Fig. 4c ). The observation of such a rapid periodic oscillation in the femoral blood velocity was entirely owed to the high time resolution of 20 ms, much shorter than the cardiac cycle of ~200 ms. The fast arterial blood flow (average speed ~4.36 cm s −1 ) passed through the entire femoral artery (length ~2 cm) within two cardiac cycles (~400 ms). At longer times post injection, the same hindlimb imaged at 39 s post injection showed full perfusion of the injected NIR-II pDA-PEG fluorescent polymer into the femoral artery ( Fig. 4d ). To further glean the oscillating blood flow front with high time resolution, we selected a region of interest of the femoral artery and analysed the NIR-II fluorescence intensity as a function of time ( Fig. 5a ). We observed evenly spaced intensity humps over a linearly increasing baseline ( Fig. 5b ), with the humps corresponding to the systolic phases of cardiac cycles of the mouse and the increasing baseline due to increased overall perfusion of pDA-PEG fluorophore into the artery vessel [3] . By subtracting the linear rise from the intensity versus time curve, we observed clear consecutive intensity spikes in the time course due to periodic ventricular ejections ( Fig. 5c ). Further, the linear-baseline-subtracted fluorescence intensity versus time was made into a movie that clearly showed the blood flow variations over the two phases of each heartbeat ( Fig. 5d–j and Supplementary Movie S2 ). The blood flow versus time showed a similar cardiogram waveform ( Fig. 5c ) as previous Doppler ultrasound measurement [37] , demonstrating that fluorescence imaging could help visualize rapid blood flow changes in real space and real time within a single cardiac cycle of the mouse. 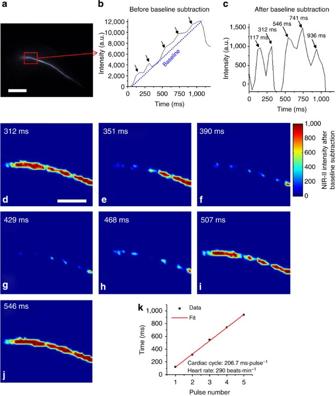Figure 5: Resolving waveform blood flow pattern with pDA. (a,b) An NIR-II fluorescence image (a) of the mouse femoral artery, where the fluorescence intensity inside the ROI red box is integrated and plotted as a function of time inb, showing an increasing profile with humps corresponding to ventricular ejections of cardiac cycles. The scale bar inaindicates 5 mm. (c) NIR-II fluorescence intensity plotted as a function of time, after a linear increasing baseline is subtracted from the plot shown inb, featuring five cardiac cycles in the plot. (d–j) Time course NIR-II fluorescence images of the red box area shown ina, after subtraction of a time-dependent linearly increasing background given by the baseline inb. Note that these seven images correspond to a complete cardiac cycle from 312 to 546 ms. SeeSupplementary Movie 2for a video showing the real-time evolution of the linear-background-subtracted fluorescence intensity. The scale bar indindicates 1 mm, which applies to all images ofd–j. (k) Time point of NIR-II fluorescence spikes corresponding to ventricular ejections shown inc, plotted over several heart pulses (black squares). The data are fitted to a linear function with its slope of 206.7 ms per pulse corresponding to the period of each cardiac cycle. Figure 5: Resolving waveform blood flow pattern with pDA. ( a , b ) An NIR-II fluorescence image ( a ) of the mouse femoral artery, where the fluorescence intensity inside the ROI red box is integrated and plotted as a function of time in b , showing an increasing profile with humps corresponding to ventricular ejections of cardiac cycles. The scale bar in a indicates 5 mm. ( c ) NIR-II fluorescence intensity plotted as a function of time, after a linear increasing baseline is subtracted from the plot shown in b , featuring five cardiac cycles in the plot. ( d – j ) Time course NIR-II fluorescence images of the red box area shown in a , after subtraction of a time-dependent linearly increasing background given by the baseline in b . Note that these seven images correspond to a complete cardiac cycle from 312 to 546 ms. See Supplementary Movie 2 for a video showing the real-time evolution of the linear-background-subtracted fluorescence intensity. The scale bar in d indicates 1 mm, which applies to all images of d – j . ( k ) Time point of NIR-II fluorescence spikes corresponding to ventricular ejections shown in c , plotted over several heart pulses (black squares). The data are fitted to a linear function with its slope of 206.7 ms per pulse corresponding to the period of each cardiac cycle. Full size image It is also interesting to note that the dots observed along the femoral artery in the baseline-subtracted images ( Fig. 5f–h ) were at fixed positions over time and corresponded to local higher NIR-II intensity regions along the femoral artery. These high-intensity local regions were found to coincide with locations along the vessel with slightly larger vessel diameters (by ~20%) of the lumen measured with the vessel image. That is, more NIR-II pDA-PEG fluorophores in the blood were filled into a larger lumen and thus exhibited higher NIR-II intensity ( Supplementary Fig. 9 ). From the NIR-II fluorescence oscillations with an average period of 206.7 ms per cardiac cycle ( Fig. 5k ), we measured a heart rate of 290 beats per minute for the mouse, which agreed with previous results via cardiac gating [38] . Thus, the high temporal and high spatial resolution NIR-II imaging afforded by the high brightness of the conjugated polymer led to remarkably rich details of blood flows and cardiac cycles in vivo . In vivo fluorescence imaging of live animals in the NIR-II region benefits from deeper penetration of up to a few millimetres inside the body and reduced scattering of photons that scales inversely proportional with wavelength as ~ λ − w ( w =0.22–1.68) in biological tissues [3] , [9] . Conjugated polymers have been widely used in organic solar cells [26] , [39] , light-emitting diodes [40] , [41] and organic electronics [42] , [43] . Fluorescent imaging with conjugated polymers has been limited to emission wavelength <900 nm [44] , [45] , [46] . Our current work developed the NIR-II agent with >1,000-nm fluorescence based on conjugated polymers for biological imaging both in vitro and in vivo [47] . The facile synthetic route of donor–acceptor copolymers could allow further tuning of the optical properties of the polymers through modifying the donor–acceptor structures ( Supplementary Fig. 10 ) and the length of the copolymer. A more electron-donating donor and a more electron-withdrawing acceptor typically result in smaller band gap of the copolymer [48] , and a longer copolymer exhibits reduced band gap due to a greater delocalization of π-electrons [30] . This could lead to a library of polymers with tunable excitation and emission wavelengths for NIR-II imaging (see Supplementary Fig. 10 for several polymers synthesized thus far). With such development, we envisage fluorophores with different emission wavelengths in the 1.0- to 1.7-μm NIR-II window, allowing for multicolour molecular imaging of different biomarkers. In addition, further improved penetration depth could be achieved in vivo by tuning the emission wavelength. A salient advantage of the pDA-PEG polymer as an NIR-II fluorophore for in vivo live animal imaging is its much higher quantum yield (~1.7%) than SWNTs (~0.4%) previously used for hindlimb blood flow tracking [3] . This allows for much faster (20-ms exposure time versus previous 100 ms) [3] video-rate imaging of dynamic changes in the blood flow labelled by NIR-II fluorophore, pushing the limit of temporal resolution to a previously unattainable level of >25 f.p.s. (the instrument frame rate limit is 50 f.p.s. due to an overhead time of 19 ms). Although the pDA-PEG polymer has similar quantum efficiency (~1.7%) to nanoparticles of small organic molecules (~1.8%) [18] , since the major peak of the small organic molecule nanoparticles is located at ~920 nm while the major peak of pDA-PEG polymer is at ~1,050 nm, the pDA-PEG polymer has a greater portion of emitted photons in the >1,000-nm NIR-II region (~70%) than the small molecule nanoparticles (~40%) [18] . Taken together, the high fluorescence quantum yield, red-shifted fluorescence emission in the NIR-II region and low density of the pDA polymer require 10~100 × lower mass dose of injection than previous NIR-II fluorophores (such as SWNTs [1] , [2] , [3] , [9] , [10] , [11] , [12] , QDs [6] , [7] , [15] , [16] , [17] , rare-earth doped nanoparticles [8] and nanoparticles incorporating organic molecules [18] ) to reach the same in vivo imaging quality, and allow for dynamic fluorescence imaging with much shorter exposure time and higher temporal resolution. This high temporal resolution well exceeds the heart rate of mice (~5 beats per second or~200 ms per cycle) by five times, eliminating the need for cardiac gating typically required for low-frame-rate cardiovascular imaging techniques [38] , [49] . Previous fluorescence imaging and tracking of blood flow usually require the removal of scattering tissue over the vessels of interest to afford higher spatial resolution and gating devices to eliminate image blurring due to cardiac and respiratory motions on a faster timescale than the temporal resolution of image acquisitions (~10 f.p.s.) [38] , [50] . Ultrasound imaging and OCT with ultrafast image acquisition rate (kHz~MHz) have shown the advantages of measuring fast blood flow and cardiac cycles [51] , [52] , [53] ; however, the spatial resolution (in the 10 μm~1 mm range) and signal-to-noise ratio are suboptimal due to long wavelengths [54] and speckles [55] , [56] . Here by utilizing NIR-II fluorescence with reduced tissue scattering and an ultrafast frame rate of >25 f.p.s., we have enabled simultaneous blood velocity and cardiac cycle measurements as well as high-resolution imaging of blood vessels 1–2 mm deep under otherwise highly scattering skin tissues [57] . We have also proved the concept that the polymer-based NIR-II fluorophores can be used to track blood flow in capillaries with sub-10 μm diameters ( Supplementary Fig. 11a ), which are well below the spatial resolutions of traditional ultrasound and OCT. On the basis of the capillary blood flow-tracking images, we measured the capillary blood velocity to be ~55.2 μm s −1 ( Supplementary Fig. 11b ), in good agreement with previous studies [58] , [59] . The dynamic range of blood velocity measurement in our NIR-II imaging system using the pDA fluorophores is derived as 0–640 mm s −1 based on the brightness of the fluorophore and the detector sensitivity ( Supplementary Note 1 ). In addition, we have shown that the pDA-PEG fluorophores can be used to track regional blood flow and redistribution as a result of increased metabolic demand after heat-induced inflammation of the tissue ( Supplementary Fig. 12 ), providing a direct diagnostic tool for visualizing the metabolic difference of the tissue. The heavy-metal-free nature of NIR-II fluorescent copolymers bodes well for potentially low-toxicity agents for in vivo applications [60] . In a cellular toxicity study, we found that the toxicity of pDA-PEG nanoparticles depended on the surfactant coating, and a surfactant with branched PEG exhibited alleviated toxicity (see Methods). The mice injected with pDA-PEG were monitored over a period of up to 2 months without showing obvious toxic effects or health problems. We also attempted tuning the size of the pDA-PEG nanoparticles and obtained the smallest pDA-PEG with an average hydrodynamic size of <6 nm ( Supplementary Fig. 13 , and also see Methods for more information). Systematic investigation is required to study the long-term fate and toxicology of pDA-PEG nanoparticles, which is beyond the scope of the current work. Real-time haemodynamic imaging could be of central importance to better understand various cardiovascular diseases and to design treatment strategies [61] . An ideal NIR-II fluorescent agent capable of achieving haemodynamic imaging with high spatial and temporal resolutions should have tunable emission wavelength in the >1,000-nm region to minimize tissue scattering, high fluorescence quantum efficiency (>5%) for ultrashort imaging exposure time. The current work opens up future research to achieve these goals and could eventually lead to NIR-II fluorescence agents suitable for clinic use. Synthesis of pDA copolymer The synthesis of monomers M1 and M2 can be found in previous publications [62] , [63] , [64] . For the synthesis of the pDA copolymer, 0.091 g of monomer M1 (0.2 mmol), 0.148 g of the monomer M2 (0.2 mmol) and 15 ml of anhydrous toluene were mixed in a two-neck flask. The solution was flushed with N 2 for 10 min, and 15 mg of Pd(PPh 3 ) 4 was added into the flask. Then the solution was flushed with N 2 for another 25 min. The two-neck flask was placed in an oil bath and heated up carefully to 110 °C. The mixture was stirred for 24 h at 110 °C under N 2 atmosphere. After the reaction was complete, the mixture was allowed to cool down to room temperature, and the polymer was precipitated by adding 100 ml of methanol and filtered through a Soxhlet thimble. Soxhlet extraction was performed with methanol, hexanes and chloroform. Eighty milligrams of the polymer were obtained as a green solid from the chloroform fraction by rotary evaporation and dried under vacuum overnight with a moderate yield of 56%. Characterizations of monomers and pDA copolymer All compounds, including the monomers M1 and M2, and the pDA copolymer, were characterized using nuclear magnetic resonance (NMR) spectroscopy. The 1 H NMR and 19 F NMR spectra were measured on a Bruker AV-400 spectrometer at room temperature. Chemical shifts were described as δ values (p.p.m. ), where tetramethylsilane was used as an internal reference. Splitting patterns were labelled as s (singlet), d (doublet), t (triplet), m (multiplet) and br (broad). As such, the NMR spectral assignments for the two monomers M1 and M2, as well as the product polymer, are given as follows: Monomer M1: 1 H NMR (400 MHz, CDCl 3 ): δ 2.95 (t, 2 H), 1.76 (m, 2 H), 1.39–1.30 (m, 10 H), 0.91 (t, 3 H). 19 F NMR (400 MHz, CDCl 3 ): −129 p.p.m. (s, Ar-F). Monomer M2: 1 H NMR (400 MHz, CDCl 3 ): δ 7.06 (s, 2 H), 4.35 (d, 4 H), 1.78 (m, 2 H), 1.37–1.70 (m, 16 H), 0.96–1.03 (m, 12 H), 0.44 (s, 18 H). Polymer pDA: 1 H NMR (400 MHz, CDCl 3 ): δ 6.80 (br, 2 H), 4.31 (br, 4 H), 3.06 (br, 2 H), 2.01–1.21 (br, 30 H), 0.81–1.21 (br, 15 H). Elemental analysis of the pDA copolymer was performed on a Flash EA 1112 elemental analyser. Elemental composition of pDA copolymer was calculated based on the molecular formula (C 41 H 53 FO 5 S 2 ) n as C: 69.26%; H: 7.80%; O: 11.25%, and compared with measured elemental composition by the elemental analyser: C, 70.08%; H, 7.73%; O, 11.09%. Molecular weight and polydispersity of the pDA copolymer were measured using gel permeation chromatography. The number-average molecular weights ( M n ), weight-average molecular weights ( M w ) and polydispersity index (PDI, M w / M n ) were determined using polystyrene as the reference. Measurements were carried out using a Waters 515 HPLC pump, a Waters 2414 differential refractometer and three Waters Styragel columns (HT2, HT3 and HT4) with THF as the eluent at a flow rate of 1.0 ml min −1 at a temperature of 35 °C. Preparation of pDA-PEG and pDA-PEG-NH 2 The as-synthesized pDA polymer was dissolved in THF at a mass concentration of 75 μg ml −1 and mixed with an aqueous solution of DSPE-mPEG(5 kDa) (1,2-distearoyl- sn -glycero-3-phosphoethanolamine- N -[methoxy(polyethyleneglycol, 5000)], Laysan Bio) at a concentration of 1.1 mg ml −1 with a 1:9 volume ratio for making the pDA-PEG, or with an aqueous solution of DSPE-PEG-NH 2 (5 kDa) (1,2-distearoyl- sn -glycero-3-phosphoethanolamine-N-[amino(polyethyleneglycol, 5000)], Laysan Bio) at 1.1 mg ml −1 with a 1:9 volume ratio for making the pDA-PEG-NH 2 . The pDA polymer remained soluble in the mixed solvent without any precipitation. Then the mixture was dialysed against water to remove THF and make a THF-free, clear aqueous solution of pDA-PEG or pDA-PEG-NH 2 polymers. To remove aggregates formed during dialysis, the suspension was ultracentrifuged for 30 min at 300,000 g and only the supernatant was retained. Free, unbound surfactant in the solution was removed through 30-kDa centrifugal filters (Amicon) without causing any instability to the pDA-PEG polymers, suggesting that the hydrophobic core of pDA and the hydrophilic shell of DSPE-mPEG were making a strongly held complex. Preparation of pDA-PEG-Erbitux bioconjugate A 200-μl solution of pDA-PEG-NH 2 after excess surfactant removal was concentrated to a mass concentration of 320 μg ml −1 , determined by a mass extinction coefficient of 30.4 l g −1 cm −1 at its peak absorbance in the UV–vis-NIR absorption spectrum. Then this solution was mixed with 1 mM sulfo-SMCC for 1 h in PBS at pH 7.4. On the other hand, 12.3 μl of Erbitux solution (Bristol-Myers Squibb) at a concentration of 2 mg ml −1 (~13.3 μM) was mixed with a 1.64 μl solution of Traut’s reagent (Sigma) at 1 mM concentration and 86 μl PBS solution. In the mixture the molar ratio of Erbitux antibody to Traut’s reagent was 1:10. The mixture of Erbitux antibody and Traut’s reagent was allowed to react for 1.5 h at room temperature. After removing excess sulfo-SMCC from the polymer solution and excess Traut’s reagent from the antibody solution by filtration through 30-kDa centrifugal filters (Amicon), the two solutions were mixed and allowed to react for 2 days in PBS at 4 °C to make the pDA-PEG-Erbitux bioconjugate. Spectral characterizations of pDA-PEG UV–vis-NIR absorption spectrum of pDA-PEG polymer in water was measured with a Cary 6000i UV–vis-NIR spectrophotometer, background-corrected for contribution from water. The measured range was 400–900 nm. The NIR-II fluorescence spectrum was taken using a home-built NIR-II spectroscopy set-up in the 900- to 1,500-nm region. The excitation source was an 808-nm diode laser (RMPC lasers) at an output power of 160 mW and was filtered by an 850-nm short-pass filter (Thorlabs), a 1,000-nm short-pass filter (Thorlabs), an 1,100-nm short-pass filter (Omega) and a 1,300-nm short-pass filter (Omega). The excitation at 808 nm was intentionally chosen to balance absorption and scattering to afford maximum penetration depth of excitation light for in vivo imaging. The excitation beam was allowed to pass through an aqueous solution of pDA-PEG polymer in a 1-mm path cuvette (Starna Cells) and the emission was collected in the transmission geometry with a 900-nm long-pass filter (Thorlabs) to reject the excitation light. The emitted fluorescence from the sample was directed into a spectrometer (Acton SP2300i) equipped with a liquid-nitrogen-cooled InGaAs linear array detector (Princeton OMA-V). The emission spectrum was corrected after raw data acquisition to account for the detector sensitivity profile and extinction feature of the filter using the MATLAB software. Determination of fluorescence quantum yield of pDA-PEG Fluorescence quantum yield of the pDA-PEG polymer in water was measured in a similar way to a previous publication [32] , using the NIR-II fluorescent IR-26 dye as the reference (quantum yield=0.5%) [31] . For reference calibration on our set-up, a stock solution of 1 mg ml −1 IR-26 dissolved in 1,2-dichloroethane (DCE) was diluted to a DCE solution with its absorbance value of ~0.10 at 808 nm. Then this sample was diluted using DCE to a series of samples with their absorbance values at 808 nm of ~0.08, ~0.06, ~0.04 and ~0.02. Using these highly diluted samples with low absorbance minimized any secondary optical processes such as re-absorption and re-emission effects. Then a total of five IR-26 solutions in DCE with linearly spaced concentrations (including the one with absorbance of ~0.10) were loaded into a 10-mm path fluorescence cuvette (Starna Cells) one at a time. The excitation source was an 808-nm diode laser (RMPC lasers) with a linewidth full-width at half-maximum of 1.89 nm at an output power of 160 mW and filtered by an 850-nm short-pass filter (Thorlabs), a 1,000-nm short-pass filter (Thorlabs), an 1,100-nm short-pass filter (Omega) and a 1,300-nm short-pass filter (Omega). The emission was collected in the transmission geometry with a 900-nm long-pass filter (Thorlabs) to reject the excitation light and the emission spectrum was taken in the 900- to 1,500-nm region. The same absorption and emission measurements were carried out for pDA-PEG polymers and SWNTs in aqueous solutions too. Then all emission spectra of both the reference and the samples were corrected after raw data acquisition to account for the detector sensitivity profile and the extinction profiles of the filters, and integrated in the 900- to 1,500-nm NIR-II region. The definition of quantum yield dictates that all emitted photons should be taken into account for quantum yield measurement [65] . In our quantum yield measurements, since an 808-nm laser is used, ideally the integration of the emission spectra should start from 809 nm to cover the complete emission band; however, due to the limited choice of excitation and emission filters, we started the integration from 900 nm, which would give an underestimated quantum yield. Nonetheless, this underestimation would not be too much since one could see from the emission spectra that the emission dropped rapidly below 950 nm, meaning there would not be too much fluorescence emission under 900 nm. The integrated NIR-II fluorescence intensity was plotted against absorbance at the excitation wavelength of 808 nm and fitted into a linear function. Two slopes, one obtained from the reference of IR-26 in DCE and the other from the sample (pDA-PEG or SWNT), were employed in the calculation of the quantum yield of the sample, based on equation (1) as follows: where n sample and n ref are the refractive indices of water and DCE, respectively. AFM imaging of pDA-PEG AFM image of pDA-PEG was acquired with a Nanoscope IIIa multimode AFM in the tapping mode. The sample for imaging was prepared by drop-drying a highly diluted aqueous solution of pDA-PEG polymer at a mass concentration of 750 ng l −1 on the SiO 2 /silicon substrate without any post-processing steps. To plot the size distribution of the pDA-PEG polymeric nanoparticles, 100 nanoparticles were measured from the AFM images and their heights were used to generate the histogram of size distribution. Owing to the effect of tip size convolution in AFM [66] , the height measurement from the AFM micrograph, rather than the lateral size measurement, was used to measure the size of the nanoparticles deposited on the substrate. Dynamic light scattering (DLS) analysis of pDA-PEG DLS was performed using a solution of pDA-PEG at 0.75 μg ml −1 in PBS in a 1-cm quartz cuvette. A PBS solution was used to mimic the ionic strength in blood because the hydrodynamic size of pDA-PEG was dependent on the ionic strength. The data were collected using a Brookhaven Instruments 90Plus Particle Size Analyzer. Cell incubation and staining All cell culture media were supplemented with 10% fetal bovine serum, 100 μg ml −1 streptomycin, 100 IU ml −1 penicillin and L-glutamine. The human glioblastoma U87-MG cells were cultured in low glucose Dulbecco’s Modified Eagle Medium, with 1 g l −1 D -glucose and 110 mg l −1 sodium pyruvate, in the presence of 5% CO 2 . Human breast cancer MDA-MB-468 cells were cultured in Leibovitz’s L-15 medium at 37 °C in absence of CO 2 . Cells were maintained in a 37 °C incubator. For cell staining, cells were trypsinized before the as-made pDA-PEG-Erbitux bioconjugate was incubated with both EGFR-positive (MDA-MB-468) and EGFR-negative (U87-MG) cell lines at a concentration of 5 μg ml −1 at 4 °C for 1 h, followed by washing the cells with 1 × PBS to remove all free, unbound pDA-PEG-Erbitux bioconjugate in the suspension. NIR-II fluorescence imaging of cancer cells Targeted cell imaging in the 1.0- to 1.7-μm NIR-II window was carried out using a 658-nm laser diode with a 150-μm-diameter excitation beam focused by a × 50 objective lens (Olympus). The NIR-II fluorescence from pDA-PEG-Erbitux bioconjugate was collected using a liquid-nitrogen-cooled, 320 × 256 pixel, two-dimensional (2D) InGaAs camera (Princeton Instruments, 2D OMA-V). The excitation light was filtered out using a 900- and a 1,000-nm long-pass filter (Thorlabs) so that the intensity of each pixel in the camera represented fluorescence in the 1.0- to 1.7-μm NIR-II region. The exposure time was 3 s for all fluorescence images. Mouse handling All vertebrate animal experiments were performed under the approval of the Stanford University’s Administrative Panel on Laboratory Animal Care. Eight-week old female BALB/c mice were obtained from Charles River and housed at the Research Animal Facility of Stanford under our approved animal protocols. Before hindlimb vessel imaging, all mice were anaesthesized in a rodent anaesthesia machine with 2 l min −1 O 2 gas flow mixed with 3% Isoflurane. Then the hair over the hindlimb skin was carefully removed using Nair to avoid causing wounds to the skin. Tail vein injection of the pDA-PEG contrast agent was carried out in dark and synchronized with the camera that started continuous image acquisition simultaneously. The injected dose was a 200 μl bolus of the pDA-PEG in a 1 × PBS solution at a mass concentration of 0.25 mg ml −1 . During the time course of imaging the mouse was kept anaesthetized by a nose cone delivering 1.5 l min −1 O 2 gas mixed with 3% Isoflurane. Ultrafast video-rate NIR-II vessel imaging Video-rate NIR-II vessel imaging was carried out in a similar manner as our previous publication [3] . In brief, imaging was carried out on a home-built imaging set-up consisting of a 2D InGaAs camera (Princeton Instruments, 2D OMA-V). The excitation was provided by an optical-fibre-coupled 808-nm diode laser (RMPC Lasers), intentionally chosen to balance absorption and scattering to afford maximum penetration depth of excitation light for in vivo imaging. The high fluorescence quantum yield of the pDA-PEG also ensured sufficient emission for ultrafast in vivo imaging despite the non-resonant excitation under 808 nm. The light was collimated by a collimator with a focal length of 4.5 mm (ThorLabs) and filtered by an 850- and a 1,000-nm shortpass filter (ThorLabs). The power density of the excitation laser at the imaging plane was 140 mW cm −2 , significantly lower than the reported safe exposure limit of 329 mW cm −2 at 808 nm [67] . The emitted fluorescence from the mouse was allowed to pass through a 900- and a 1,000-nm long-pass filter (Thorlabs) and to be focused on the InGaAs detector by a lens pair consisting of two NIR achromats (200 and 75 mm; Thorlabs). The distance between the two NIR achromats was adjusted to have only one hindlimb of the mouse included in the field of view. The camera was set to expose continuously using the LabVIEW software with an exposure time of 20 ms. NIR-II images were acquired with a frame rate of 25.6 f.p.s. due to a 19-ms overhead time during readout. In vitro toxicity study of pDA-PEG We determined the in vitro toxicity of pDA-PEG by MTS assay using a CellTiter96 kit (Promega) on human breast cancer MDA-MB-468 cells. To evaluate how the surfactant coating of the pDA polymer affected the nanoparticles’ in vitro toxicity, we coated the pDA polymer (the same formulation as in Fig. 1 ) with DSPE-mPEG and poly(maleic anhydride-alt-1-octadecene)methoxy(polyethyleneglycol, 5 kDa) (C18-PMH-mPEG), respectively, where DSPE-mPEG has one linear PEG chain, while C18-PMH-mPEG has many branched PEG chains. For in vitro toxicity study, ~5,000 MDA-MB-468 cells were incubated per well with 100 μl of Leibovitz’s L-15 medium spiked with pDA-DSPE-mPEG or pDA-C18-PMH-mPEG at serially diluted concentrations ( n =6 for each concentration). The cells were kept at 37 °C in a humidified atmosphere for 36 h in the absence of CO 2 . MDA-MB-468 cell medium (100%) without any pDA-PEG was taken as the positive control, while MDA-MB-468 cell medium spiked with 20 μM Doxil was taken as the negative control. Immediately before addition of 15 μl of CellTiter96 for the colorimetric assay, the polymer-spiked medium was removed from each well in the plate and replaced with fresh MDA-MB-468 cell growth medium. This would prevent any interference in the absorbance readings from the intrinsic colour of pDA-PEG. After 1.5 h, the colour change was quantified using a plate reader, which took absorbance readings at 485 nm. Cell viability was plotted as a fraction of the absorbance value of the positive control wells incubated without any pDA-PEG after baseline subtraction of the absorbance for medium alone. The negative control wells had an average cell viability value of ~60% after 36 h of incubation, which was as expected. We found from the in vitro toxicity study that pDA-DSPE-mPEG has a half maximal inhibitory concentration (IC50) level of ~30 μg ml −1 , while pDA-C18-PMH-mPEG has an IC50 level of >150 μg ml −1 . The pDA-PEG solution could not be further concentrated to an even higher concentration, preventing us from measuring the cell viability under an incubation concentration of >150 μg ml −1 . It is also noteworthy that the linear or branched PEG coating did not alter the fluorescence quantum efficiency to a noticeable level. Hydrodynamic size tuning of pDA-PEG nanoparticles The hydrodynamic size tuning was performed by coating the pDA polymer with surfactants of different PEG molecular weights (2 and 5 kDa) and changing the initial pDA concentration in the THF solution (0.025–0.075 mg ml −1 ; please see the ‘Preparation of pDA-PEG and pDA-PEG-NH 2 ’ section in Methods) before mixing with 1.1 mg ml −1 DSPE-mPEG in water. After the pDA-PEG nanoparticles were made in each synthesis condition, DLS analysis was performed to evaluate each sample’s hydrodynamic diameter as a function of initial pDA concentration in the THF solution and the molecular weight of PEG in the surfactant (please see the ‘Dynamic light scattering (DLS) analysis of pDA-PEG’ section in Methods). The dependence of pDA-PEG hydrodynamic size on initial pDA concentration and PEG molecular weight is plotted in Supplementary Fig. 13 , showing that both smaller PEG and lower initial concentration of pDA favour the formation of smaller pDA-PEG nanoparticles in aqueous solution. However, it is noteworthy that DLS was not able to discriminate the ‘empty’ nanoparticles without any pDA molecules loaded inside, and therefore the size distribution of the measured hydrodynamic diameters below ~4 nm could be due to the micelles formed by the DSPE-mPEG surfactants only. How to cite this article: Hong, G. et al. Ultrafast fluorescence imaging in vivo with conjugated polymer fluorophores in the second near-infrared window. Nat. Commun. 5:4206 doi: 10.1038/ncomms5206 (2014).